A magneto-electro-optical effect in a plasmonic nanowire material Electro- and magneto-optical phenomena play key roles in photonic technology enabling light modulators, optical data storage, sensors and numerous spectroscopic techniques. Optical effects, linear and quadratic in external electric and magnetic field are widely known and comprehensively studied. However, optical phenomena that depend on the simultaneous application of external electric and magnetic fields in conventional media are barely detectable and technologically insignificant. Here we report that a large reciprocal magneto-electro-optical effect can be observed in metamaterials. In an artificial chevron nanowire structure fabricated on an elastic nano-membrane, the Lorentz force drives reversible transmission changes on application of a fraction of a volt when the structure is placed in a fraction-of-tesla magnetic field. We show that magneto-electro-optical modulation can be driven to hundreds of thousands of cycles per second promising applications in magneto-electro-optical modulators and field sensors at nano-tesla levels. Dynamic control of metamaterials promises a radical expansion of photonic functionalities. The use of superconductors, phase change and nonlinear media, liquid crystals, carrier injection, graphene and coherent control [1] , [2] , [3] , [4] has been reported to achieve tuneable electromagnetic properties. Microwave magnetoelastic metamaterials [5] , Terahertz MEMS metamaterials [6] , [7] , [8] , [9] , [10] and optical reconfigurable metamaterials driven by thermal expansion [11] and Coulomb forces [12] have been realized. Several phenomena that allow the modulation of optical material properties with external electric or magnetic fields are known. We first recall the well-known linear electro-optical or Pockels effect of changing or inducing birefringence of crystals in the presence of static electric field E that is used in numerous light-modulation applications. In terms of the field-induced correction to the dielectric tensor ɛ ij it may be introduced as . Another example is the electro-optical Kerr effect that is normally observed in isotropic liquids and manifests itself as birefringence proportional to the square of applied electric field: . Linear magneto-optical effects, i.e. the optical Faraday effect that induces circular birefringence and dichroism for transmission along a longitudinal magnetic field H and the polar, longitudinal and transversal magneto-optical Kerr effects that are usually observed for reflected waves, are well-known and applications include optical isolators and reading magnetically stored information with reflected light, (ref. 13 ). The quadratic magneto-optical effect of inducing optical birefringence by transverse magnetic field is also well documented and known as the Voigt effect in gases and the Cotton–Mouton effect in solids and liquids, (refs 14 , 15 ). Also known in the literature are phenomena of electro- and magneto-gyration that describe changes of optical activity in chiral media in the presence of electric and magnetic fields [16] , [17] and a nonreciprocal optical magneto-electric effect, leading to directional birefringence and dichroism [18] , [19] , [20] , [21] , [22] . Here we report the observation of a magneto-electro-optical effect that manifests itself as strong changes of optical properties of a metamaterial in response to simultaneous application of external electric and magnetic fields and does not depend on reversal of the propagation direction of the wave. It may be described by the following term in the constitutive equation: Magneto-electro-optical nanowire metamaterial To create a metamaterial exhibiting strong magneto-electric changes of its optical response, we designed a flexible plasmonic nanostructure that can be reconfigured by the Lorentz force on simultaneous application of external electric E and magnetic H fields, see Fig. 1 . To engage the Lorentz force, we used a continuous conductive chevron nanowire array of length L along which we applied electric voltage V to introduce an electric field | E |= V / L and a current I that is necessary for the appearance of the Lorenz force, F = L I × H . The chevron pattern was chosen as it has good longitudinal elasticity due to its spring-like structure, while providing plasmonic optical resonances, continuous electrical paths that can support currents and simplicity in terms of nanofabrication. 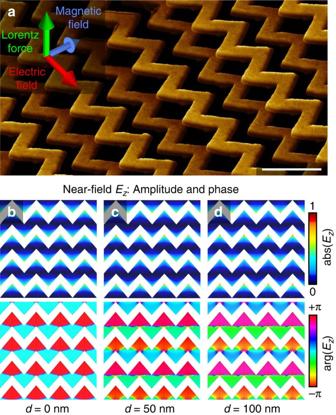Figure 1: Lorentz magneto-electro-optical metamaterial. (a) Artistic impression of the nanostructure of current-carrying flexible chevron strips that are driven by the Lorentz force. The scale bar, 1 μm. (b–d) To illustrate reconfiguration-induced changes of the plasmonic response of the nanostructure, we show the magnitude and phase of the near-fieldEzperpendicular to the plane of the metamaterial, 10 nm above the chevron strips. This field component is linked to the light-induced oscillating charge separation in the gold layer. The effect of displacing every second nanowire can be seen in both amplitude and phase patterns, most dramatically in the latter: the increasing displacementdfrom (b) 0 to (c) 50 and (d) 100 nm leads to a growing phase difference between alternating rows. In these field maps, the nanowires are separated by white areas and the first and third complete chevron strips are being displaced. Incident light is at the wavelength of 1,550 nm and linearly polarized with the electric field perpendicular to the nanowires. Figure 1: Lorentz magneto-electro-optical metamaterial. ( a ) Artistic impression of the nanostructure of current-carrying flexible chevron strips that are driven by the Lorentz force. The scale bar, 1 μm. ( b – d ) To illustrate reconfiguration-induced changes of the plasmonic response of the nanostructure, we show the magnitude and phase of the near-field E z perpendicular to the plane of the metamaterial, 10 nm above the chevron strips. This field component is linked to the light-induced oscillating charge separation in the gold layer. The effect of displacing every second nanowire can be seen in both amplitude and phase patterns, most dramatically in the latter: the increasing displacement d from ( b ) 0 to ( c ) 50 and ( d ) 100 nm leads to a growing phase difference between alternating rows. In these field maps, the nanowires are separated by white areas and the first and third complete chevron strips are being displaced. Incident light is at the wavelength of 1,550 nm and linearly polarized with the electric field perpendicular to the nanowires. Full size image Optical properties of metallic nanostructures, such as the metamaterial investigated here, are determined by the localized plasmonic response of coupled oscillations of conduction electrons and the electromagnetic near field induced by the incident light. The near-field distribution and thus the plasmonic response are highly sensitive to the geometry of the structure. Therefore, changes on the nanometric scale, that are induced by the action of the Lorentz force, can have a strong effect on the nanostructure’s optical properties. This is illustrated by Fig. 1b–d using somewhat exaggerated levels of displacement (for clarity): the electric field distribution in the near-field of the structure changes dramatically on out-of-plane movement of every second nanowire of the array. The magneto-electro-optical effect appears concurrently with thermally-induced changes of the optical properties that are driven by the release of Joule heat in the nanostructure. This thermo-optic effect appears even in the absence of the external magnetic field and is not sensitive to the current direction. In the first approximation, it is proportional to the power dissipated in the array and thus to | I | 2 ∼ V 2 ∼ | E | 2 . As the nanowire material used in our experiments was non-magnetic, we observed no optical response on application of the external magnetic field H alone. In our experiments, we targeted the magneto-electro-optical response in the near-infrared part of the spectrum, at telecom frequencies. The metamaterial reported here is an array of separated gold nanowires of length L =35 μm manufactured on a 50-nm-thick silicon nitride membrane that was cut into separate elastic chevron strips with 770 nm chevron period (see Methods and Fig. 2 ). The nanowire strips form a regular grid with pitch of 775 nm. Alternating nanowires were electrically connected to terminals on both ends, so that electric field applied across the metamaterial array induces a current I in every second strip. Optical transmission of the metamaterial has plasmonic resonances in the near infrared, see Fig. 2b . 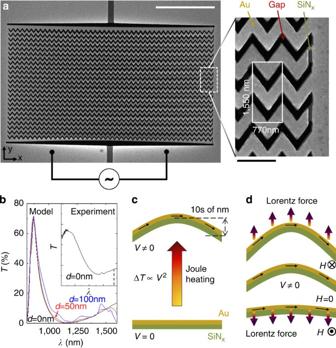Figure 2: Lorentz and thermal forces in reconfigurable metamaterial. (a) Scanning electron microscopy image showing the metamaterial device with chevron nanowires. The white scale bar, 10 μm, the black scale bar in the inset, 1 μm. (b) TransmissionTof the nanostructure as a function of wavelengthλfor several displacementsd. Experimental results and numerical simulations are plotted on identical scales and the wavelength used in the modulation experiments is marked by a dashed line. (c) Electro-thermal and elastic forces compete in the bimorph nanowire consisting of gold (yellow) and silicon nitride (green) when an applied voltageVleads to a temperature increase ΔTdue to Joule heating. (d) Current in a magnetic fieldHproduces a Lorentz force competing with the thermal effect. Figure 2: Lorentz and thermal forces in reconfigurable metamaterial. ( a ) Scanning electron microscopy image showing the metamaterial device with chevron nanowires. The white scale bar, 10 μm, the black scale bar in the inset, 1 μm. ( b ) Transmission T of the nanostructure as a function of wavelength λ for several displacements d . Experimental results and numerical simulations are plotted on identical scales and the wavelength used in the modulation experiments is marked by a dashed line. ( c ) Electro-thermal and elastic forces compete in the bimorph nanowire consisting of gold (yellow) and silicon nitride (green) when an applied voltage V leads to a temperature increase Δ T due to Joule heating. ( d ) Current in a magnetic field H produces a Lorentz force competing with the thermal effect. Full size image In the presence of external magnetic field H , nanowires that bear current are subject to the Lorentz force F = L I × H that moves them from the plane of the array against the elasticity force to a maximum displacement of few tens of nanometres, see Fig. 2d . In the reconfigurable metamaterial with anchored ends of the strips, the Lorentz force leads to homogeneous displacement at the centre that contributes most to the modulation of optical properties of the metamaterial. This deformation changes the electromagnetic coupling between neighbouring nanowires and thus the plasmonic response of the array at optical frequencies. At zero displacement, symmetry dictates identical light-induced charge oscillations in all chevron strips, see Fig. 1b . With displacement of every second strip, charges in neighbouring strips oscillate with an increasing phase difference and with lower (higher) amplitude in repositioned (stationary) strips, see Fig. 1c,d . In general, the Lorentz force-induced change of the optical properties has components that are even and odd functions of the nanowire displacement along the z -direction. Indeed, if initially all strips are located in the plane of the membrane, any change of optical properties is insensitive to the direction of displacement z . However, if alternated nanowires are pre-displaced in the z -direction, the change in the optical properties will be sensitive to the direction of displacement z . The out-of-plane motion of every second strip increases the nanostructure's periodicity perpendicular to the strips, so that the metamaterial's unit cell in the dynamic regime is 770 × 1,550 nm. Strictly speaking, for the metamaterial to be an effective medium film, that is, to transmit and reflect light without scattering, the optical wavelength shall be longer than the unit cell in all directions. Characterization of the sample was performed at the edge of the effective medium regime of the deformed structure at the telecommunications wavelength of 1,550 nm. Therefore, our results shall be interpreted as indication on what changes in permittivity ɛ of a hypothetical homogeneous medium shall be obtained to reach the same modulation depth as the actual nanostructure. Experimental characterization of the effect To detect the magneto-electro-optical effect, we characterized transmission changes of the metamaterial induced by simultaneous application of the electric and magnetic fields. The magneto-electro-optical effect and the thermo-optical effect can be effectively separated by changing the magnetic field strength. Moreover, with a harmonically modulated external electric control signal the thermal mechanism will respond at the doubled frequency of modulation due to its quadratic nature. However, the Lorentz mechanism will create a modulated optical response at the control frequency. Results for non-zero values of the magnetic field strength are presented on Fig. 3 . It shows the optical modulation depth recorded at the frequency f for different amplitudes and frequencies of the control signal V = A cos(2 πft ). A high-frequency zoom-up displays the resonant feature. Correspondingly, Fig. 4 shows the optical modulation depth as a function of control signal amplitude A and magnetic field H at characteristic frequencies of modulation. 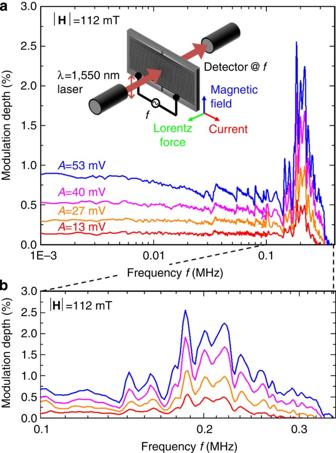Figure 3: Magneto-electro-optical modulation. Modulation of transmission with an external electrical control signal of amplitudeAat different frequenciesfin a static magnetic fieldH. Transmission modulation is detected at the frequency of electric modulation. Figure 3: Magneto-electro-optical modulation. Modulation of transmission with an external electrical control signal of amplitude A at different frequencies f in a static magnetic field H . Transmission modulation is detected at the frequency of electric modulation. 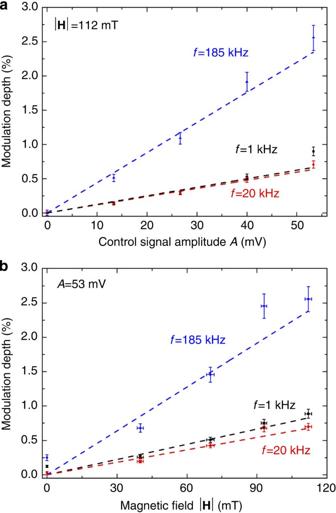Figure 4: Magneto-electro-optic effect. Linear relation between transmission change and applied external control signals detected at selected modulation frequenciesf. Transmission modulation as a function of (a) electric modulation amplitude for a |H|=112 mT static magnetic field and (b) magnetic field for a fixed electric modulation amplitude ofA=53 mV (|E|=1.5 kV m−1). Error bars show the s.d. and dashed lines are linear fits through the origin. Full size image Figure 4: Magneto-electro-optic effect. Linear relation between transmission change and applied external control signals detected at selected modulation frequencies f . Transmission modulation as a function of ( a ) electric modulation amplitude for a | H |=112 mT static magnetic field and ( b ) magnetic field for a fixed electric modulation amplitude of A =53 mV (| E |=1.5 kV m −1 ). Error bars show the s.d. and dashed lines are linear fits through the origin. Full size image The results clearly indicate a linear dependence of the sample's transmissivity on the external magnetic and electric fields and this can be described as linear magneto-electro-optical effect . The effect has a clear resonant nature (a peak at about 200 kHz) that is related to the mechanical resonance of the chevron nanowires that are supported at both ends. Off-resonance the effect is weakly dependent on the frequency of modulation. The effect is enabled by the Lorentz force acting against the elasticity of the membrane. Indeed the modulation vanishes at zero magnetic field. Based on the nanostructure's resistance of R =27 Ω, a voltage of V =53 mV leads to I s = V /(12 R )=160 μA current in each of the 12 electrically connected strips, corresponding to a maximum Lorentz force of F s = LI s | H |=640 pN per strip in our experiments when | H |=112 mT magnetic field is applied. The proportionality of the effect to the driving voltage seen in Fig. 4 is only possible if the ‘hot’ nanowires bearing the current are pre-displaced from the plane of the membrane. We argue that such displacement results from post-fabrication bow-type deformation of the sample and/or is induced by the Joule heating of the bimorph nanowires. Indeed, the equilibrium temperature of the heated strips is proportional to power dissipation. The dissipated power at V =53 mV is V 2 / R =100 μW, corresponding to about 40 K temperature increase at current-carrying nanowire centres compared with their ends. Such temperature increase will cause few tens of nanometres static strip displacement due to differential thermal expansion of gold and silicon nitride [23] . In contrast, Fig. 5a shows the optical modulation depth recorded at frequency 2 f at zero magnetic field H for different amplitudes A and frequencies f of the control signal V . Correspondingly, Fig. 5b shows the optical modulation depth as a function of control signal amplitude A at characteristic frequencies of modulation. The results show a quadratic dependence of the sample’s transmissivity change on the external electric field, which shall be expected for the thermo-optic effect. Similar to the magneto-electro-optical contribution, the effect has a peak at the mechanical resonance of the metamaterial. Off-resonance, the effect progressively rolls off with the frequency of modulation. Indeed, the thermo-optical effect depends on heating and cooling of the nanostructure, which is controlled by conductive heat transport from the nanowires to the surrounding membrane and then to the supporting silicon frame. Our calculations starting from the law of heat conduction and published values for the thermal properties of 50-nm-thick films of gold [24] and silicon nitride [25] predict a characteristic roll-off frequency of few tens of kilohertz, which is consistent with the experimentally observed roll-off ( Fig. 5 ). 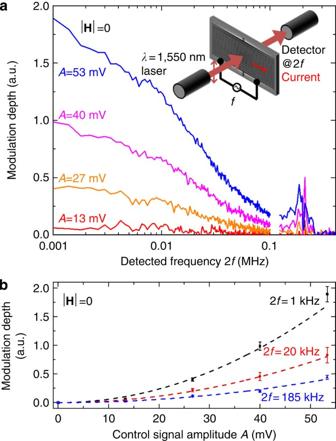Figure 5: Thermal modulation. Transmission modulation with an external electrical control signal at different frequencies without magnetic field. Detection at twice the frequency of modulation 2f. Modulation depth as a function of (a) frequency and (b) electrical modulation amplitude. Error bars show the s.d. and dashed lines are quadratic fits through the origin. Figure 5: Thermal modulation. Transmission modulation with an external electrical control signal at different frequencies without magnetic field. Detection at twice the frequency of modulation 2 f . Modulation depth as a function of ( a ) frequency and ( b ) electrical modulation amplitude. Error bars show the s.d. and dashed lines are quadratic fits through the origin. Full size image We are not aware of any highly flexible natural media structured on the nanoscale with distinctly anisotropic conductivity that could exhibit a similar magneto-electro-optical effect. Therefore our work is a further illustration of the power of the metamaterial paradigm to create materials with novel properties. In the past this included negative optical magnetism [26] , negative refraction [27] , asymmetric transmission [28] , toroidal resonances [29] , as well as extremely high nonlinear [30] and electro-optical coefficients [12] . Here we extend this to the observation of a magneto-electro-optical effect that has never been observed before. We note that Lorentz force based MEMS magnetic field sensors have been reported [31] , [32] , but cannot be approximated as effective media. From our experimental data, we can estimate the order of magnitude of χ (3) in as χ (3) / n ∼ 10 −4 (m V −1 T −1 ), where n is the refractive index. We note that a nonreciprocal optical magneto-electric effect is also known. It results from bi-anisotropic constitutive equations that have terms mixing the polarization (magnetization) of the medium with the magnetic field (electric field) of the wave at optical frequencies, resulting in a dependence of the effect on the propagation direction of the wave [18] , [19] , [20] , [21] , [22] . The phenomenon observed here is different: in the constitutive equation it results only from the term that describes the change of the dielectric tensor in response to the slowly variable externally applied electric and magnetic fields, which control the deformation of the nanostructure. Such change therefore does not depend on the wave propagation direction, and therefore leads to a reciprocal effect. Control experiments confirm within experimental accuracy that the effect is the same for opposite directions of wave propagation, see Table 1 . Table 1 Reciprocity of the magneto-electro-optical effect. Full size table Both lateral uniformity and magnitude of the observed optical effect can be improved by thinning the chevron nanowires at their ends, which will lead to larger and more uniform displacement of the more rigid central part of the pattern, as has been suggested in ref. 33 . The use of stronger currents and magnetic fields will lead to stronger Lorentz force and larger displacements of the strips, but the Joule heat dissipation and inelastic deformation of the nanostructure will limit the parameter field in which reversible and reproducible changes and consistent signal modulation can be achieved. The main obstacle in achieving higher modulation depth will be thermal damage to the device that we expect to fail at a few hundred millivolts of driving signal. Displacements and optical modulation can also be increased by using longer nanowires to increase the elasticity of the structure and by using more elastic membranes. A considerable increase in the amplitude of high-frequency resonant responses can be attained by reducing the damping associated with the ambient air in which the nanowires move, thus placing the metamaterial in a vacuum cell will help to increase the Q -factor of the response. Furthermore, the design of the plasmonic resonators can be optimized and their spacing reduced to couple them more strongly, increasing the sensitivity of optical properties to nanoscale displacements. In conclusion, we observe a magneto-electro-optical effect that is driven by the Lorentz force acting on an array of nanowires. Already the effect in the chevron nanowire array can be used for magnetic field-sensing applications, where availability of the second control parameter (the electric field) can be exploited to engage highly sensitive zero balance phase detection techniques to realize sensitivity at nano-Tesla levels. Moreover, we argue that a dedicated optimization of the metamaterial design can lead to the observation of stronger effects suitable for practical application in light-modulation devices. Reconfigurable photonic metamaterial fabrication The reconfigurable nanostructure was fabricated from a 50-nm-thick low stress silicon nitride membrane, which is 500 × 500 μm 2 in size and supported by a silicon frame. A 50-nm-thick gold layer was thermally evaporated onto the membrane and structured with a focused ion beam system (FEI Helios 600 NanoLab), with the contact electrodes connected to a source measurement unit (Keithley 2636) through a vacuum feedthrough for in situ electrical characterization. Using focused ion beam milling, the chevron pattern was milled through both gold and silicon nitride layers, creating both the plasmonic resonators and the supporting suspended silicon nitride strips in one step. Then the terminals at the strip ends were electrically separated by removing the gold film in selected areas. The overall size of the metamaterial array is 35 × 20 μm. Experimental and numerical characterization In the numerical simulations shown in Figs 1b–d and 2b and the optical experiments presented in Figs 2 , 3 , 4 , 5 , the nanostructure was illuminated from the silicon nitride side with the optical electric field polarized perpendicular to the strips. High-frequency modulation was studied with a 1,550 nm laser transmitted through the nanostructure, while modulating the electric signal applied to the metamaterial using a signal generator and applying static magnetic fields with neodymium magnets. The modulated signal was detected by an InGaAs photodetector (New Focus 1811) and two lock-in amplifiers (Stanford Research SR830 up to 100 kHz and SR844 >100 kHz). The numerical simulations are full three-dimensional Maxwell calculations based on a finite element method solver (Comsol). One unit cell consisting of a chevron pair was modelled with periodic boundary conditions. How to cite this article : Valente, J. et al . A magneto-electro-optical effect in a plasmonic nanowire material. Nat. Commun . 6:7021 doi: 10.1038/ncomms8021 (2015).